Unfolding a molecular trefoil derived from a zwitterionic metallopeptide to form self-assembled nanostructures While used extensively by nature to control the geometry of protein structures, and dynamics of proteins, such as self-organization, hydration forces and ionic interactions received less attention for controlling the behaviour of small molecules. Here we describe the synthesis and characterization of a novel zwitterionic metallopeptide consisting of a cationic core and three distal anionic groups linked by self-assembling peptide motifs. 2D NMR spectra, total correlated spectroscopy and nuclear Overhauser effect spectroscopy, show that the molecule exhibits a three-fold rotational symmetry and adopts a folded conformation in dimethyl sulfoxide due to Coulombic forces. When hydrated in water, the molecule unfolds to act as a self-assembling building block of supramolecular nanostructures. By combining ionic interactions with the unique geometry from metal complex and hydrophobic interactions from simple peptides, we demonstrate a new and effective way to design molecules for smart materials through mimicking a sophisticated biofunctional system using a conformational switch. Protein folding [1] , [2] , [3] , [4] is an essential step in generating a functional protein. Partial unfolding of natively folded proteins often results in fibrillar structures or filaments that play important roles in either normal physiological functions [5] or pathological states [6] , [7] . For example, Pepys et al . [8] discovered that amyloidogenic intermediates of lysozyme consist of a partially unfolded conformers. Hurle et al . [9] have shown that the conversion of an immunoglobulin light chain into amyloid proceeds via partial unfolding under acidic conditions. Recently, partially unfolding α-lactalbumin has found application in cancer therapy [10] . Although these proteins differ in sequence and native folds, their fibrils are morphologically and structurally similar, implying similar mechanisms of unfolding and fibrillation. These studies, in addition to providing useful insights for understanding pathogenic fibrillogenesis and contributing to the development of potential therapeutics, also offer fundamental guiding principles for designing soft materials as a new class of biomimetics [11] , [12] , [13] , [14] , [15] . The structures of amyloid fibrils have been determined in atomic details [16] , [17] , [18] , [19] , [20] , the partial unfolding of proteins to form fibrillar structures exhibits several distinctive common features. First, the folding–unfolding transition requires a flexible molecular architecture. Second, the polypeptide backbone and hydrophobic side chains are largely buried within the folded structure. Partial unfolding exposes the hydrophobic groups, and fibrillation provides an alternative means of sequestering those groups from solvent. Third, the forces governing protein conformation include those resulting from intramolecular (hydrogen bonding and salt bridge formation), and intermolecular (solvent–solvent and solvent–protein) interactions. Both types of interactions depend on the specific structure of the protein and on the nature of the solvent [21] , [22] , [23] . Changing the nature of the solvent can change the balance between the driving forces for folding versus unfolding [22] , [23] , [24] , potentially destabilizing the native folded structure [24] , [25] , and initiating the self-assembly of fibrillar structures. The fibrillation conditions for a wide range of proteins, correlates with charge, secondary structure and hydration. Despite being well-established in the field of protein structures [26] or applied in design of hybrid system and crystalline materials [27] , [28] , [29] , [30] , these guiding principles received less attention in the design of soft materials made of small molecules. Thus, we aim to apply these interactions for designing biomimetic materials. Here we describe the synthesis and characterization of a trefoil zwitterioinic metallopeptide designed to mimic the folding/unfolding behaviour of proteins. The hydration of the ionic species separates the charges in the zwitterions, and results in the unfolding of the trefoil, and by removing the hydration force the trefoil folds back. Such a folding–unfolding conformational transition leads to the exposure of the hydrophobic arms of the trefoil molecule, thus favouring intermolecular self-assembly in its unfolded conformation. Furthermore, we find that the self-assembly of this trefoil molecule is pH responsive. The pH of the solvent modulates the trefoil molecule’s hydration, which, in turn, is implicated in interfibrillar interactions that control filament morphology. This simple multimodular molecular system mimics protein unfolding in precise molecular details, and opens new possibilities for developing simple small molecules that mimic the behaviour and ultimately the functions of the complex biological systems. 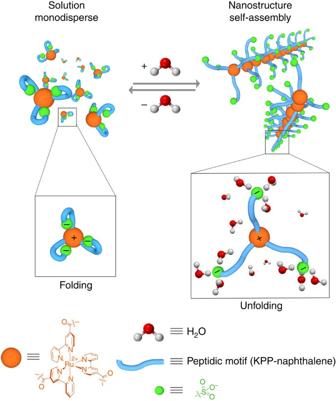Figure 1: Reversible unfolding of a trefoil molecule by hydration force for self-assembly. A trefoil molecule, consisting of a positive charged core (that is, [Ru(II)(bpy)3]2+analogue) and three negative charged groups (that is, sulfonate) that are covalently linked by three peptidic arms Lys-Phe-Phe-naphthalene (KPP-naphthalene), exists as a folded monomer in DMSO due to self-charge compensation (for clarity, Na+is not shown). The addition of water hydrates the ions in the trefoil molecule and unfolds it to allow the formation of supramolecular nanofibrils through intermolecular self-assembly. By decreasing the percentage of water using blowing air, nanofibrils dissociate. The trefoil molecules fold back and stay as monomers. Molecular design Figure 1 shows the concept of molecular design. The molecule consists of three modules, a dicationic metal complex as the positively charged core, three tripeptide arms [31] capped by sulfonate groups as the distal anions [32] . To generate a molecule capable of forming a three-dimensional folded structure, we choose an octahedral [Ru(II)(bpy) 3 ] 2+ complex [33] as the core because ruthenium (II) also has a high affinity for sulfonate [34] . Since Hunter and colleagues successfully used octahedral [Zn(II)(bpy) 3 ] 2+ to create a molecular trefoil knot [35] , the [Ru(II)(bpy) 3 ] 2+ should also permit the formation of an open trefoil. To ensure the flexibility of the tripeptide arms for the folding–unfolding switch, we connected the metal complex to the peptide through the side chain of the lysine residue rather than the peptide main chain. To allow sufficient separation of the anions and the cationic core, we arrange the sulfonate groups at the end of the peptidic backbone. Overall, this molecule possesses a three-fold rotational symmetry and relies on the balance between ionic interactions and hydration force to determine the preferred molecular conformation. We expected that this arrangement would facilitate a conformational switch when the dielectric constant of the solvent changes. Figure 1: Reversible unfolding of a trefoil molecule by hydration force for self-assembly. A trefoil molecule, consisting of a positive charged core (that is, [Ru(II)(bpy) 3 ] 2+ analogue) and three negative charged groups (that is, sulfonate) that are covalently linked by three peptidic arms Lys-Phe-Phe-naphthalene (KPP-naphthalene), exists as a folded monomer in DMSO due to self-charge compensation (for clarity, Na + is not shown). The addition of water hydrates the ions in the trefoil molecule and unfolds it to allow the formation of supramolecular nanofibrils through intermolecular self-assembly. By decreasing the percentage of water using blowing air, nanofibrils dissociate. The trefoil molecules fold back and stay as monomers. Full size image Synthesis of trefoil zwitterionic metallopeptide According to the molecular design, we synthesize the trefoil molecule 5 in three primary steps as presented in Fig. 2 . We first prepare the peptide motif 1 using solid-phase peptide synthesis. On peptide motif 1 , N - tert -butoxycarbonyl (Boc) group protects the ε-amino group of the lysine residue to facilitate the direct coupling of taurine to the peptide main chain. Following the coupling reaction, N -Boc deprotection in trifluoroacetic acid/dichloromethane mixture affords compound 2 , the peptide with sulfonate group at its C-terminal, in 95% yield. An organometallic chelation of the bipyridine ligand ( 3 ) and dichloro( p -cymene)Ru(II) dimer in dimethylformamide (DMF) under reflux condition produces octahedral Ru-complex 4 as the positive charged core. After purification by Sephadex column chromatography, we obtain pure complex 4 as a red powder in a 62% yield. It takes 24 h to complete the final step of the synthesis—the direct coupling of 2 and 4 assisted by HBTU ( O -(benxotriazol-1-yl)- N , N , N′ , N′ -tetramethyluronium hexafluorophosphate) and DIEA ( N , N -diisopropylethylamine) in DMF at 60 °C. Following a two-step purification, Sephadex column chromatography and semi-preparative HPLC, we obtain the trefoil molecule 5 as an orange powder in 46% yield. 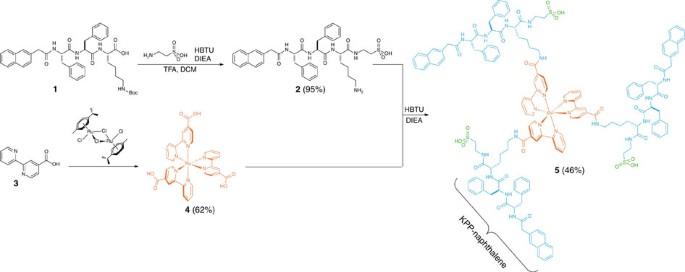Figure 2: Synthesis of the trefoil complex5based on octahedral-coordinated Ru(II). Compound1is coupled with taurine followed by removal of the Boc protecting group with trifluoroacetic acid in dichloromethane to give2. The reaction of3with dichloro(p-cymene)Ru(II) dimer produces complex4. Being assisted by HBTU and DIEA in anhydrous DMF, the coupling reaction of2and4affords the trefoil complex5(the metal complex core is represented in orange, the peptidic motif KPP-naphthalene in blue, and the sulfonate in green). Figure 2: Synthesis of the trefoil complex 5 based on octahedral-coordinated Ru(II). Compound 1 is coupled with taurine followed by removal of the Boc protecting group with trifluoroacetic acid in dichloromethane to give 2 . The reaction of 3 with dichloro( p -cymene)Ru(II) dimer produces complex 4 . Being assisted by HBTU and DIEA in anhydrous DMF, the coupling reaction of 2 and 4 affords the trefoil complex 5 (the metal complex core is represented in orange, the peptidic motif KPP-naphthalene in blue, and the sulfonate in green). Full size image Folded structure We investigate the structure of trefoil molecule 5 in dimethylsulphoxide (DMSO; 4.0 mM) using 1D 1 H nuclear magnetic resonance ( 1 H NMR), and 2D 1 H-total correlation spectroscopy (TOCSY) and 1 H-nuclear Overhauser effect spectroscopy (NOESY). The combination of 1D 1 H NMR ( Supplementary Fig. 1 ) and 2D 1 H-TOCSY ( Supplementary Fig. 2 ) data provides the complete 1 H NMR resonance assignments ( Supplementary Table 1 ). 800 MHz 1 H NMR ( Supplementary Fig. 1 ) provides sufficient dispersion of the NH signals (W 1 , W 2 , W 4 and W 7 in the region of 7.92–8.27 p.p.m.) and splittings of C–H signals (X 2 , quartet, X 4 and X 7 are triplets of doublets), simplifying resonance assignments. The protons 1a and 1b are assigned on the basis of 1 H-TOCSY cross peaks with the W 1 proton. The protons 3a, 3b and 3c are assigned on the basis of cross peaks with the W 2 and X 2 protons. Following that, the proton 3d is assigned based on the cross peak with 3a, 3b and 3c protons. On the basis of the cross peak with the 3d proton, the proton W 3 is assigned. The combination of chemical shifts, peak splits, and cross peaks allows the assignment of protons 5b, 6b, 6c, 6d, 6e and 8a. On the basis of the cross peak with 8a, proton Z 8 is assigned. The remaining aromatic C–H protons are assigned to the region between 7.29–7.13 p.p.m. After completing the assignments of protons, we identified the nuclear Overhauser effects (NOEs; Supplementary Table 1 , Supplementary Figs 2 and 3 ) to use as distance restraints for structural calculations. By applying energy minimization in Chem3D, we build up the 3D structure of 5 based on the crystal structure of [Ru(II)(bpy) 3 ] 2+ derivative [36] and observed NOEs for 5 . NOEs between 3a/1b, 3d/1a, 3d/1b, W 1 /3a, W 1 /3b and W 1 /X 2 indicate the proximity between the taurine residues and the side chain of lysine residues on the trefoil molecule. In particular, the NOEs between 1a, 1b and 3d restrict the relative conformations of these residues. We assigned the phenylalanine main chain adjacent to lysine residue based on the NOE between W 4 and 1b. The NOE between Z 4 and W 7 restricts the main chain conformation of the second phenylalanine residue. Finally, the NOE between Z 8 and W 4 restricts the conformation of the acetyl naphthalene moiety. The cross peaks between the aromatic C–H protons in the region of 8.30–7.30 p.p.m. define the relative positions of all the aromatic rings of the molecule. 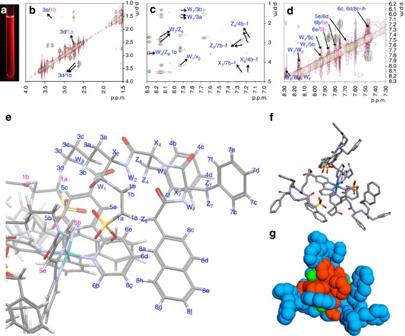Figure 3: 3D molecular structure of5in DMSO based on 2D NMR spectra. (a) Optical image of5in DMSO-d6in NMR tube under Ultraviolet light (on the right of the NMR tube). Overlapped spectra of1H-TOCSY (green) and1H-NOESY (red) (b), (c) and (d) assigned with NOEs. (e) Assignment of protons on a stick model of5in DMSO (inter-ligand NOEs are signed in magenta). (f) Full stick model and (g) space-filling model (colour representations of different portion of the molecule corresponding to the chemical structure inFig. 2) of5in DMSO. Figure 3e (stick model), 3 f (stick model without protons) and 3 g (space-filling model) show a 3D structure of trefoil 5 calculated by energy minimization that satisfies all distance restraints. Clearly, molecule 5 adapts a folded structure in DMSO. Since the low pK a (1.5) of taurine’s sulfonic acid group ensures the moiety is negatively charged in neutral condition, this folded structure is likely due to the three sulfonate anions remaining in close proximity to the positive charged ruthenium centre. Figure 3: 3D molecular structure of 5 in DMSO based on 2D NMR spectra. ( a ) Optical image of 5 in DMSO- d 6 in NMR tube under Ultraviolet light (on the right of the NMR tube). Overlapped spectra of 1 H-TOCSY (green) and 1 H-NOESY (red) ( b ), ( c ) and ( d ) assigned with NOEs. ( e ) Assignment of protons on a stick model of 5 in DMSO (inter-ligand NOEs are signed in magenta). ( f ) Full stick model and ( g ) space-filling model (colour representations of different portion of the molecule corresponding to the chemical structure in Fig. 2 ) of 5 in DMSO. Full size image Unfolded structure To explore the structure of the trefoil molecule 5 under self-assembling conditions, we performed 1D 1 H NMR, 2D 1 H-TOCSY and 1 H-NOESY of the molecule in DMSO/D 2 O (2/1) mixture (4.0 mM). Note that the NMR signals are only slightly broader under the modified solvent conditions, so the observed species in NMR are not polymeric. However, the fluorescence scattering of DMSO/D 2 O solution of 5 ( Fig. 4a ; the ultraviolet light is placed on the right side of the NMR tube) indicates the formation of aggregates. This is confirmed by the high-resolution transmission electron microscopy (HRTEM) image of the dispersion that reveals uniform fibrils with widths of 4.5±0.1 nm ( Fig. 4b ). In the 1D 1 H NMR spectrum ( Supplementary Fig. 4 ), all NH protons disappear because of D 2 O exchange. Comparison of the 2D 1 H-TOCSY ( Supplementary Fig. 5 ) and 1 H-NOESY spectra ( Supplementary Fig. 6 ) shows fewer inter-residue NOEs ( Fig. 4d , Supplementary Table 2 ) of 5 under self-assembly conditions. While the lack of NOE-based distance restraints does not rule out the existence of folded conformers under conditions of self-assembly, the decreased spectral dispersion and increased degeneracy of diastereotopic proton signals ( Fig. 4c ) indicates that discrete folded conformations are less favoured under these conditions. Combining this information with excluded volumes due to steric interactions, we propose that trefoil 5 adopts an unfolded conformation ( Fig. 4e,f ) with maximum length of 34.2 Å under conditions that lead to self-assembly of single molecule stacking for fibrils with width of 4.5±0.1 nm [31] . We also observed upfield shifts of protons (1a and 1b; Fig. 4c ) in the vicinity of the sulfonate groups and downfield shifts of all the other protons ( Supplementary Fig. 4 ) after introducing D 2 O into the system. These shifts agree with the unfolding of 5 . 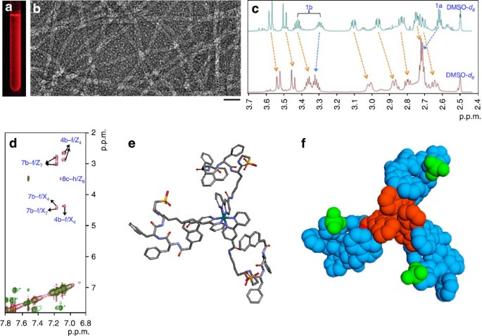Figure 4: 3D molecular structure of5in DMSO and D2O mixture based on 2D NMR spectra. (a) Optical image of5in DMSO-d6/D2O (2/1) in NMR tube under Ultraviolet light (on the right of the NMR tube). (b) HRTEM of the mixture in NMR tube of Figure a. (c)1H NMR spectra of5in DMSO (cyan) and in DMSO/D2O (2/1; dark red) indicate the upfield shift of protons close to sulfonate. (d) Overlapped spectra of1H-TOCSY (green) and1H-NOESY (red) with assignment of NOEs. (e) Stick model and (f) space-filling model (colour representation is same as inFig. 2) of5in DMSO-d6/D2O. Figure 4: 3D molecular structure of 5 in DMSO and D 2 O mixture based on 2D NMR spectra. ( a ) Optical image of 5 in DMSO- d 6 /D 2 O (2/1) in NMR tube under Ultraviolet light (on the right of the NMR tube). ( b ) HRTEM of the mixture in NMR tube of Figure a. ( c ) 1 H NMR spectra of 5 in DMSO (cyan) and in DMSO/D 2 O (2/1; dark red) indicate the upfield shift of protons close to sulfonate. ( d ) Overlapped spectra of 1 H-TOCSY (green) and 1 H-NOESY (red) with assignment of NOEs. ( e ) Stick model and ( f ) space-filling model (colour representation is same as in Fig. 2 ) of 5 in DMSO- d 6 /D 2 O. Full size image Self-assembly and pH modulation On the basis of the unfolded 3D structure of 5 in the mixed aqueous medium, multiple forces potentially contribute to the self-assembly of 5 , including hydration, electrostatics and hydrophobic interactions. These various contributions can be modulated by altering the pH. The sulfonate groups of 5 are ionisable and exist predominantly in the negatively charged form (-SO 3 − ) at pH values above the p K a . The hydration of the sulfonate group obviously depends on its ionization state (that is, the sulfonate anion is more strongly hydrated than the neutral sulfonic acid [37] , [38] ). Thus, changing pH will effectively modulate both the hydration and electrostatics of 5 . We evaluated the hydrogelation of 5 (4 mM) in water from pH 14 to 1 and use transmission electron microscopy (TEM) to examine the nanostructures formed. As shown in Fig. 5a , 5 is able to form red hydrogels at basic to neutral pH. Acidic pH condition causes syneresis, with collapse of the hydrogel and eventual suspension. The decrease in the water-carrying capacity of 5 under conditions of low pH suggests an increase in the intermolecular hydrophobic interactions. The circular dichroism spectra ( Supplementary Fig. 9 ) of 5 (4 mM) in water indicate the beta -sheet formation at basic to acidic pH, and higher pH favours beta -sheet formation. 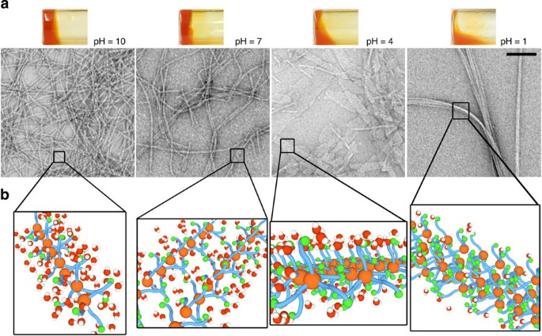Figure 5: The morphological change of the assemblies of5upon pH modulation. (a) Optical images and TEM images of5in water (4 mM) at different pH with morphology change (scale bar, 100 nm). (b) Illustration of the enhanced hydration level and negative charges of sulfonate groups by increasing pH results in multiple self-assembled morphologies. Figure 5: The morphological change of the assemblies of 5 upon pH modulation. ( a ) Optical images and TEM images of 5 in water (4 mM) at different pH with morphology change (scale bar, 100 nm). ( b ) Illustration of the enhanced hydration level and negative charges of sulfonate groups by increasing pH results in multiple self-assembled morphologies. Full size image The morphologies of the nanostructures revealed by the TEM images ( Fig. 5a ) support the hydrogelation behaviours of 5 in water as a function of pH. The TEM images obtained as a function of gelation time also reveals a two-stage cooperativity [39] in the self-assembly of 5 . Initially, self-assembly of 5 in water results in similar uniform fibrils with 5±1 nm widths regardless of pH ( Supplementary Fig. 7 ). The pH-dependent transformation of nanofibres to other morphologies occurs after an incubation period (for example, 48 h; Supplementary Fig. 8 ). At pH 10, the self-assembled fibrils observed after aging are the same as those seen initially, so no secondary rearrangement occurs. At pH 7, the fibrils maintain a uniform width but become shorter than the fibrils observed initially (or after aging at pH 10). Some fibrils append to each other, indicating increased interfibrillar interactions. At pH 4, the nanofibres transform into rectangular lamellar structure with 19–87±1 nm in width and a few micrometres in length. When the pH reaches 1, the separated uniform nanofibres transform into intertwined fibrils bundles. Apparently, the uniform nanofibres are the kinetically favoured morphology at the initial stage of self-assembly of 5 . The pH-dependent morphologies reached after aging appear to be thermodynamically stable. The uniform long fibrils formed under basic conditions are more flexible than other self-assembled morphologies of 5 at neutral or acidic pH. Since the fibrils are negatively charged under the basic conditions, the interfibrillar repulsive interactions favour thin split nanofibrils, which results in a softer hydrogel. As the pH decreases, the sulfonate groups are progressively protonated (-SO 3 H), decreasing interfibrillar repulsion, thus allowing greater interfibrillar interaction that contributes to the distribution of less tunable (shorter) fibrils and increased interfibrillar contact, as revealed in the TEM images ( Fig. 5a ). At pH 4, the collapse of the gel agrees with the transformation of fibrils to lamellar structures ( Fig. 5a ). The formation of such morphology leads to a significant reduction of the surface that is exposed to the aqueous medium compared with the nanofibres. At pH 1, nanofibres transform into the most compact morphology observed. Decreases in both the surface area available for solvent interactions and the corresponding hydration of the surface due to increased intermolecular hydrophobic interactions likely contribute to the syneresis of the hydrogel at low pH. These results illustrate that changing pH can modulate the interactions between fibrils by perturbing the balance between the electrostatic repulsion and hydrophobic interactions, thus resulting in different dominant morphologies at different pH values ( Fig. 5b ). This observation agrees with the mechanism elucidated by Boden et al . [12] , [13] , that is, multilevel of intermolecular and interfibrillar interactions dictate the morphology of the self-assembled nanostructures. Although bottom-up molecular engineering has been extensively applied in biomimetic design, the execution of polymorphism through an integrated molecular system still remains as a great challenge in materials science. To achieve this goal, fully understanding not only the individual building blocks but also the path from simplicity to complexity and efficient manipulation of molecular structure are required. By describing the design and synthesis of a trefoil zwitterionic metallopeptide that mimics the conformational transitions of proteins, we present a successful case of biomimetic folding dynamics of proteins. The elucidation of conformation transition and polymorphic self-assembly of the molecule through conventional techniques, 2D NMR, and TEM offers molecular-level insights on mechanisms of formation of self-assembled nanostructures. This research as a contribution to the exploration of polymorphism of molecular arrangements will provide insights for understanding the multiple molecular interactions that associated with the disease-causing amyloids. The polymorphic self-assembly of the trefoil molecule by pH modulation will also contribute to the understanding of the heterogeneous pHs in a cellular setting for producing polymorphic aggregates of proteins and peptides. Overall, this study provides valuable information on designing single molecular systems for exploring the conformational switch with high precision [40] . NMR spectroscopy The NMR sample of 5 without self-assembly was prepared by adding 10 mg of 5 and 500 μl DMSO- d 6 into an NMR tube and mixing them well. The NMR sample of 5 with self-assembly was prepared by dissolving 10 mg of 5 in 333 μl DMSO- d 6 in an NMR tube NMR tube, followed by the addition of 167 μl D 2 O for well mixing. The NMR spectra were recorded on a Bruker Avance NMR spectrometer operating at 800.13 MHz ( 1 H) and equipped with TCI cryoprobe and pulse-field gradients. Experiments used for sequential resonance assignments include 1 H-TOCSY, and 1 H-NOESY. All experiments were performed at 298 K. NMR data were processed using TOPSPIN (Bruker Biospin Inc.) and the data were analysed using TOPSPIN and MestReNova. Gelation test A small glass vial was charged with 5.73 mg compound 5 and 500 μl deionized water. The mixture was sonicated for dissolving. Trace amount of concentrated nitric acid or sodium hydroxide solution was added into the mixture for pH modulation. The final mixture was sonicated until mixed well. High-resolution transmission electron microscopy HRTEM micrographs were obtained with TITAN 80–300 FEG scanning transmission electron microscope by the negative-staining method with uranyl acetate solution (2%) as the staining reagent. Transmission electron microscopy TEM images were acquired by conventional TEM technique. The specimen was prepared by placing a droplet of solution/hydrogel of 5 onto a holey carbon-coated copper grid. After negative-stained with uranyl acetate solution (2%), the grid was allowed to air dray. TEM characterization was performed using a Morgani 268 transmission electron microscope. How to cite this article : Zhang, Y. et al . Unfolding a molecular trefoil derived from a zwitterionic metallopeptide to form self-assembled nanostructures. Nat. Commun. 6:6165 doi: 10.1038/ncomms7165 (2015).